Herpes simplex virus enhances chemokine function through modulation of receptor trafficking and oligomerization Glycoprotein G (gG) from herpes simplex virus 1 and 2 (HSV-1 and HSV-2, important human neurotropic pathogens) is the first viral chemokine-binding protein found to potentiate chemokine function. Here we show that gG attaches to cell surface glycosaminoglycans and induces lipid raft clustering, increasing the incorporation of CXCR4 receptors into these microdomains. gG induces conformational rearrangements in CXCR4 homodimers and changes their intracellular partners, leading to sustained, functional chemokine/receptor complexes at the surface. This results in increased chemotaxis dependent on the cholesterol content of the plasma membrane and receptor association to Src-kinases and phosphatidylinositol-3-kinase signalling pathways, but independent of clathrin-mediated endocytosis. Furthermore, using electron microscopy, we show that such enhanced functionality is associated with the accumulation of low-order CXCR4 nanoclusters. Our results provide insights into basic mechanisms of chemokine receptor function and into a viral strategy of immune modulation. The highly prevalent pathogens Herpes simplex virus type 1 and 2 (HSV-1 and HSV-2, respectively) establish latency in the peripheral nervous system and cause a variety of diseases from cold sores to encephalitis [1] , [2] . The different outcomes of HSV infection depend on the interplay between the virus and the immune system. One of the strategies of immune modulation mediated by herpes viruses consists of the expression of viral chemokine-binding proteins (vCKBP), secreted proteins that bind chemokines with high affinity [3] . All vCKBPs described to date inhibit the biological function of chemokines [4] . The sole exception is glycoprotein G (gG) from HSV-1 and HSV-2 (gG1 and gG2, respectively), which increases chemokine-mediated cell migration and signalling [5] . The lack of gG expression in HSV-1 leads to virus attenuation in mouse models of infection [6] , [7] , [8] but there are no reports addressing the role of gG in HSV-2 infections. Modulation of chemokine activities by gG may contribute to HSV-1 and HSV-2 pathogenesis. Chemokines are chemotactic cytokines that modulate cell activation and orchestrate leukocyte recruitment to the sites of injury or infection. Alterations in the chemokine network are in the onset and development of cancer, autoimmunity and neuroinflammatory diseases [9] , [10] . Chemokines are presented by glycosaminoglycans (GAGs) to specific G-protein-coupled receptors (GPCRs), triggering a variety of biological responses. Among the chemokines modulated by HSV gG is CXCL12, which binds to the ubiquitous CXCR4 receptor. The CXCL12/CXCR4 axis regulates HIV infection, plays relevant roles in the immune and nervous systems and is involved in multiple pathological conditions [11] . Chemokine receptor internalization is tightly controlled since it regulates the amount of available receptor and thereby chemokine-triggered responses [12] . Although clathrin-dependent mechanisms govern the internalization of most chemokine receptors, lipid rafts are also involved in GPCR trafficking as well as in the internalization of other types of receptors, integrins and viruses [13] . Lipid rafts are highly dynamic entities that aggregate forming larger structures, such as those located at the leading edge of migrating cells. These specialized platforms allow an optimal spatial interaction between ligands, receptors and signalling partners, and thus are believed to be pivotal for processes such as migration, lymphocyte activation and viral infection [14] , [15] . Our previous work identified HSV gG as the first vCKBP that enhances the function of chemokines in vitro and in vivo through an unknown mechanism [5] . Here, we show that secreted gG (SgG) from HSV binds to GAGs at the cell surface triggering the stabilization of functional chemokine/receptor complexes in specific microdomains of the plasma membrane, leading to a cholesterol-dependent increase of chemotaxis and signalling. Furthermore, we find a direct association between the enhanced responsiveness to chemokines and an increased nanoclustering of CXCR4 at the surface of SgG-stimulated cells. These findings strengthen our understanding of a novel immunomodulatory strategy exerted by human herpes viruses, and provide relevant insights into the biology of chemokines and their receptors. HSV SgG binds to cell surface GAGs We have previously shown that recombinant secreted HSV-1 and HSV-2 gG (SgG1 and SgG2, respectively) interact with chemokines through their GAG-binding domain without inhibiting chemokine binding to the GPCR [5] . We hypothesized that SgG could interact with the plasma membrane to modulate chemokine interaction with the GPCR. Viral protein binding to plasma membrane was detected by immunofluorescence and flow cytometry assays using human primary monocytes and CHO cells ( Fig. 1a,b,e,f , respectively). Upon CXCL12 stimulation at 37 °C, both SgG2 and CXCR4 showed significant co-localization at one of the cell edges ( Fig. 1a , bottom row, and Supplementary Fig. 1a ), whereas no changes in receptor redistribution were evident at 4 °C ( Fig. 1b ). 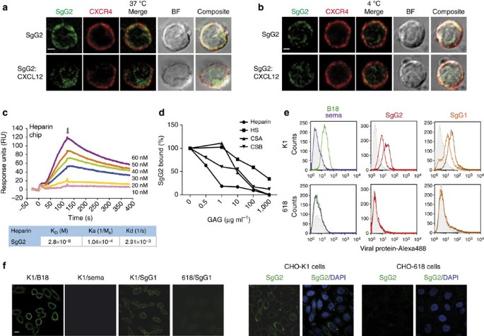Figure 1: SgGs interact with GAGs at the cell surface. (a,b) SgG2 binding to the surface of human primary monocytes. Freshly isolated monocytes were incubated with SgG2 alone or in the presence of CXCL12 at 37 °C (a) or 4 °C (b). SgG2 and endogenous CXCR4 were detected using specific polyclonal antibodies. BF, bright field images. Scale bar, 2 μm. (c) Sensorgram depicting the interaction between SgG2 and heparin by SPR. SgG2 was injected at different concentrations over biotinylated-heparin immobilized on a chip. The arrow indicates the end of the injection. All curves were analysed with the BIAevaluation software and kinetic parameters for the SgG2–heparin binding are shown in the inset table. (d) SgG2 interacts with other sulfated GAGs. SgG2, alone or in combination with increasing concentrations of the soluble heparin, heparan sulfate (HS) and chondroitin sulfate A (CS A) or B (CS B), was injected over the BIAcore chip coated with heparin. The percentage of SgG2 bound respective to protein binding in the absence of soluble GAG was plotted as a function of the concentration of each competitor GAG. (e) Binding of SgG2 (100 and 500 ng, light and dark red histograms, respectively) and SgG1 (400 and 600 ng, orange and brown histograms, respectively) to CHO cells. The viral proteins were incubated with wild-type CHO-K1 cells (upper row) or GAG-deficient CHO-618 cells (lower row) during 30 min at 4 °C and surface-bound proteins were detected by flow cytometry. Vaccinia virus (VACV) B18 and ectromelia virus (ECTV) sema were used as positive and negative controls, respectively (left histograms). (f) Immunofluorescence experiment showing binding of SgG1, SgG2 or the control proteins VACV B18 and ECTV sema to the surface of CHO cells. Proteins were stained with an anti-SgG1 monoclonal antibody, an anti-gG2 polyclonal antibody or anti-His antibodies, and DNA was stained with DAPI. Scale bar, 10 μm. All assays shown are representative of at least two independent experiments. Figure 1: SgGs interact with GAGs at the cell surface. ( a , b ) SgG2 binding to the surface of human primary monocytes. Freshly isolated monocytes were incubated with SgG2 alone or in the presence of CXCL12 at 37 °C ( a ) or 4 °C ( b ). SgG2 and endogenous CXCR4 were detected using specific polyclonal antibodies. BF, bright field images. Scale bar, 2 μm. ( c ) Sensorgram depicting the interaction between SgG2 and heparin by SPR. SgG2 was injected at different concentrations over biotinylated-heparin immobilized on a chip. The arrow indicates the end of the injection. All curves were analysed with the BIAevaluation software and kinetic parameters for the SgG2–heparin binding are shown in the inset table. ( d ) SgG2 interacts with other sulfated GAGs. SgG2, alone or in combination with increasing concentrations of the soluble heparin, heparan sulfate (HS) and chondroitin sulfate A (CS A) or B (CS B), was injected over the BIAcore chip coated with heparin. The percentage of SgG2 bound respective to protein binding in the absence of soluble GAG was plotted as a function of the concentration of each competitor GAG. ( e ) Binding of SgG2 (100 and 500 ng, light and dark red histograms, respectively) and SgG1 (400 and 600 ng, orange and brown histograms, respectively) to CHO cells. The viral proteins were incubated with wild-type CHO-K1 cells (upper row) or GAG-deficient CHO-618 cells (lower row) during 30 min at 4 °C and surface-bound proteins were detected by flow cytometry. Vaccinia virus (VACV) B18 and ectromelia virus (ECTV) sema were used as positive and negative controls, respectively (left histograms). ( f ) Immunofluorescence experiment showing binding of SgG1, SgG2 or the control proteins VACV B18 and ECTV sema to the surface of CHO cells. Proteins were stained with an anti-SgG1 monoclonal antibody, an anti-gG2 polyclonal antibody or anti-His antibodies, and DNA was stained with DAPI. Scale bar, 10 μm. All assays shown are representative of at least two independent experiments. Full size image We checked whether HSV gG interacted with the cell surface through GAGs, as shown for other vCKBPs [16] , [17] . SgG2 interacted with heparin with high affinity, as demonstrated by surface plasmon resonance (SPR, Fig. 1c ) and heparin–sepharose bead pull-down assays ( Supplementary Fig. 1b ). SgG2–heparin binding was competitively inhibited by heparan sulfate and chondroitin sulfate A and B, indicating that SgG2 interacts with different GAGs with variable affinities ( Fig. 1d ). Moreover, SgG bound to wild-type CHO-K1 cells, but not to mutant CHO-618 cells deficient in GAG expression [18] confirming the relevance of GAGs in the interaction of SgG with the cell surface, as determined by flow cytometry ( Fig. 1e ) and immunofluorescence ( Fig. 1f ). As a control for positive or no binding to GAGs, we used vaccinia virus B18 and ectromelia virus sema proteins, respectively [19] ( Fig. 1e,f ). We also tested virus-free supernatants from HSV-2-infected cultures, containing secreted gG2. HSV-1 gG is not secreted during infection [20] . gG2 present in supernatants of HSV-2-infected cells bound CHO-K1. However, protein binding dropped with CHO-618 cells ( Supplementary Fig. 1c ). SgG1 also bound to the cell surface through GAGs as determined by flow cytometry and immunofluorescence ( Fig. 1e,f ). SgG2 modifies CXCR4 trafficking and prevents internalization CXCR4 internalization is not required for signalling, but it serves as a regulatory mechanism to control the strength and duration of cellular responses to CXCL12 (ref. 12 ). We investigated the effect of SgG2 on CXCR4 trafficking. SgG2 reduced CXCL12-promoted internalization of CXCR4 in MM-1 and HEK-293T cells, leading to a significant increase of CXCR4 at the surface ( Fig. 2a,d , respectively). The effect was more pronounced when the cells were pre-incubated with SgG2 before stimulation with CXCL12 ( Fig. 2a , SgG2F–CXCL12 condition) in comparison with cells stimulated with the SgG2:CXCL12 complex, suggesting that SgG2 modified cell membrane receptor trafficking independently of the presence of the chemokine. SgG1 was also capable of blocking chemokine-induced internalization of CXCR4 in Jurkat T cells ( Fig. 2b ). 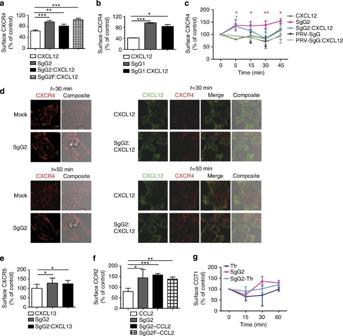Figure 2: HSV SgGs modify GPCR trafficking and upregulate the level of chemokine receptors at the cell surface. Effect of (a) SgG2 and (b) SgG1 on CXCR4 surface levels in MM-1 and Jurkat cells, respectively. SgG2F:CXCL12 indicates cells that were incubated with SgG2 for 30 min before the addition of the chemokine. In all the cases, cells were stimulated for 30 min with 1.5 μM SgG, 15 nM CXCL12 or SgG:CXCL12 at a 100:1 molar ratio, and surface receptor levels were detected by flow cytometry. (c) Amount of CXCR4 at the surface of primary human monocytes. Primary monocytes were mock treated or stimulated with 15 nM CXCL12, 750 nM SgG2 or PRV–SgG, or SgG2:CXCL12 and PRV–SgG:CXCL12 at a 50:1 molar ratio for different time points and CXCR4 surface levels were detected by flow cytometry. Plot shows two independent assays performed in triplicates. (d) Analysis of CXCL12 and CXCR4 localization by time-lapse video microscopy of ACP-CXCR4 expressing HEK-293T cells that were mock treated or stimulated with 800 nM SgG2, 8 nM CXCL12 or the complex SgG2:CXCL12 at a 100:1 molar ratio. Selected frames corresponding to the time when the movie started (t=30 min) and 20 min later (t=50 min) are shown. Scale bar, 10 μm. (e) Expression of CXCR5 at the cell surface of m300-19 B cells. Leukocytes were stimulated with 15 nM chemokine, 1.5 μM SgG2 or the complex SgG2:chemokine at a 100:1 molar ratio for 15 min. (f) Expression of CCR2 at the surface of MM-1 cells. Cells were stimulated with 5 nM CCL2, 500 nM SgG2 or a combination of CCL2 and SgG2 at a 1:100 ratio for 15 min. SgG2F:CCL2 indicates cells that were incubated with SgG2 for 30 min before the addition of the chemokine. (g) Surface expression of CD71 measured by flow cytometry in MM-1 cells on stimulation with 1 mg ml−1transferrin (Tfr), 1.5 μM SgG2 or both. In all the cases, plots show one assay run in triplicates representative of at least three independent assays unless indicated. The expression of the receptors at the surface was represented as the percentage of the value obtained for mock-treated cells at each time point. Data show mean±s.d. One-tailed unpairedt-test, *P<0.05, **P<0.01, ***P<0.001. Figure 2: HSV SgGs modify GPCR trafficking and upregulate the level of chemokine receptors at the cell surface. Effect of ( a ) SgG2 and ( b ) SgG1 on CXCR4 surface levels in MM-1 and Jurkat cells, respectively. SgG2F:CXCL12 indicates cells that were incubated with SgG2 for 30 min before the addition of the chemokine. In all the cases, cells were stimulated for 30 min with 1.5 μM SgG, 15 nM CXCL12 or SgG:CXCL12 at a 100:1 molar ratio, and surface receptor levels were detected by flow cytometry. ( c ) Amount of CXCR4 at the surface of primary human monocytes. Primary monocytes were mock treated or stimulated with 15 nM CXCL12, 750 nM SgG2 or PRV–SgG, or SgG2:CXCL12 and PRV–SgG:CXCL12 at a 50:1 molar ratio for different time points and CXCR4 surface levels were detected by flow cytometry. Plot shows two independent assays performed in triplicates. ( d ) Analysis of CXCL12 and CXCR4 localization by time-lapse video microscopy of ACP-CXCR4 expressing HEK-293T cells that were mock treated or stimulated with 800 nM SgG2, 8 nM CXCL12 or the complex SgG2:CXCL12 at a 100:1 molar ratio. Selected frames corresponding to the time when the movie started ( t =30 min) and 20 min later ( t =50 min) are shown. Scale bar, 10 μm. ( e ) Expression of CXCR5 at the cell surface of m300-19 B cells. Leukocytes were stimulated with 15 nM chemokine, 1.5 μM SgG2 or the complex SgG2:chemokine at a 100:1 molar ratio for 15 min. ( f ) Expression of CCR2 at the surface of MM-1 cells. Cells were stimulated with 5 nM CCL2, 500 nM SgG2 or a combination of CCL2 and SgG2 at a 1:100 ratio for 15 min. SgG2F:CCL2 indicates cells that were incubated with SgG2 for 30 min before the addition of the chemokine. ( g ) Surface expression of CD71 measured by flow cytometry in MM-1 cells on stimulation with 1 mg ml −1 transferrin (Tfr), 1.5 μM SgG2 or both. In all the cases, plots show one assay run in triplicates representative of at least three independent assays unless indicated. The expression of the receptors at the surface was represented as the percentage of the value obtained for mock-treated cells at each time point. Data show mean±s.d. One-tailed unpaired t -test, * P <0.05, ** P <0.01, *** P <0.001. Full size image A delay in chemokine-triggered internalization and a significant increase in surface receptor levels were also observed in human primary monocytes in the presence of SgG2, but not of pseudorabies virus (PRV)–SgG, a vCKBP that inhibits chemokine function [21] ( Fig. 2c ). Next, we analysed CXCR4 trafficking in live cells by time-lapse video microscopy using HEK-293T cells stably expressing CXCR4 engineered with a tag derived from the acyl carrier protein (ACP) [22] . The receptor constitutively trafficked in the mock-stimulated cells, whereas some areas of CXCR4 accumulation were observed at the cell surface upon SgG2 treatment ( Fig. 2d ). Incubation with CXCL12 reduced the amount of CXCR4 at the surface over time. In contrast, stimulation with the CXCL12:SgG2 complex led to a sustained presence of the receptor at the surface ( Fig. 2d ). Internalizing vesicles containing CXCR4 and CXCL12 were readily observed upon treatment with the chemokine alone ( Supplementary Movie 1 ), whereas they were much scarcer in cells stimulated with the SgG2:CXCL12 complex, where spots of chemokine and receptor were stabilized at the surface ( Supplementary Movie 2 ). A quantitative analysis showed a significant increase of CXCL12 in the proximity of CXCR4 when the chemokine was bound to SgG2 ( Supplementary Fig. 2a ). After an acidic wash, which removes surface-bound but not internalized CXCL12, less intracellular CXCL12 was observed in the SgG2:CXCL12-treated cells, in agreement with a sustained presence of CXCR4/CXCL12 at the cell surface upon SgG2 exposure ( Supplementary Fig. 2b ). We next addressed whether the effect of SgG2 on trafficking was CXCR4 specific by analysing the trafficking of two chemokine receptors, CXCR5 and CCR2. SgG2 significantly increased CXCR5 levels at the cell surface when compared with the CXCL13 control ( Fig. 2e ). SgG2 also enhances CXCL13-mediated chemotaxis [5] . Interestingly, although SgG2 neither binds nor potentiates the chemotactic properties of CCL2 (ref. 5 ), we also observed a significant increase in CCR2 levels at the cell surface on stimulation with the viral protein, in comparison with CCL2-treated cells ( Fig. 2f ). This latter result indicates that both modification of receptor trafficking and chemokine binding are required to enhance chemokine activity. However, contrary to what was observed for these GPCRs, SgG2 did not significantly modify the internalization of CD71 or transferrin receptor ( Fig. 2g ). SgG2 promotes the incorporation of CXCR4 into lipid rafts We next asked whether SgG2 could modulate the plasma membrane localization of CXCR4 using Jurkat cells transduced with the fluorescent lipid raft marker Lck 10 mCherry [23] , [24] . Neither mock-treated nor CXCL12-stimulated cells showed high co-localization values between endogenous CXCR4 and lipid rafts ( Fig. 3a ). On the other hand, SgG2 alone or the complex SgG2:CXCL12 significantly increased the presence of CXCR4 in Lck 10 mCherry-enriched domains, whereas PRV–SgG did not ( Fig. 3a ). Focal clusters of Lck 10 mCherry were observed only upon SgG2 stimulation in regions where no membrane ruffling was apparent ( Supplementary Fig. 3a ). The SgG2-induced clustering of lipid rafts and the enrichment of CXCR4 in these domains were dependent on the cholesterol content of the plasma membrane, since both effects were abrogated when cells were pretreated with the cholesterol-depleting agent methyl-beta-cyclodextrin (MβCD) ( Fig. 3a and Supplementary Fig. 3a , lower rows). Further evidence of the SgG2-promoted effect on lipid rafts and CXCR4 redistribution to these microdomains was obtained from western blot analysis of cell membrane fractions isolated according to their lipid raft content ( Fig. 3b ). SgG2 enhanced CXCR4 incorporation into lipid raft-enriched membrane fractions, in comparison with both mock- or CXCL12-stimulated Jurkat cells. LCK mostly localized to lipid raft membrane fractions after activation with CXCL12. Interestingly, an increase in the lipid raft-associated protein LCK as well as the ganglioside GM1 in the fractions corresponding to lipid raft-rich membranes was also apparent upon SgG2 stimulation of the cells. This demonstrated that GM1 and LCK maintain a lipid raft localization after exposure to SgG2. These effects correlated with the SgG2-mediated increase in lipid raft clustering and GM1 surface staining observed in our microscopy studies ( Supplementary Fig. 3a and Supplementary Fig. 4a ). In addition, SgG2 increased CXCL12 co-localization with the fluorescent Lck 10 mCherry lipid raft marker in cells, suggesting that the complex SgG2:CXCL12 preferentially binds to lipid raft-associated CXCR4 ( Supplementary Fig. 2c ). 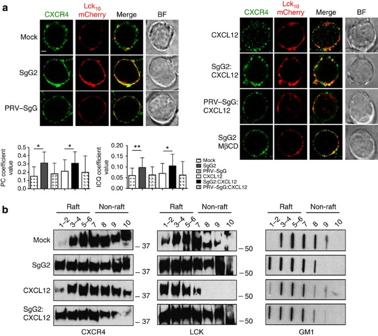Figure 3: SgG2 promotes clustering of lipid rafts and incorporation of CXCR4 to these microdomains. (a) Quantitative analysis of lipid rafts and CXCR4 co-localization. Jurkat T cells were transduced with the fluorescent lipid raft marker Lck10mCherry (in red), incubated with CXCL12 alone or in combination with SgG2 or PRV–SgG, and stained for endogenous CXCR4 (shown in green). Representative images from two independent assays are shown. The intensity correlation analysis (ICA) method was utilized to quantify co-localization of the fluorescent signals. As a result, two coefficients were calculated: Pearson’s coefficient (PC), which varies from −1 (perfect inverse correlation) to +1 (perfect positive correlation), and intensity correlation quotient (ICQ), which provides an overall index of whether the intensities are associated in a dependent or segregated manner (−0.5≤ICQ≤+0.5). Bar plots show PC and ICQ coefficient values obtained from 14 to 20 cells for a region of interest (ROI) corresponding to the entire plasma membrane. SgG2-induced focal clustering of lipid rafts and CXCR4 incorporation into these domains following cholesterol extraction with MβCD is also shown (lower row). BF, bright field. Scale bar, 2 μm. Data show mean±s.d. Two-tailed unpairedt-test, *P<0.05, **P<0.01 (b) Analysis of CXCR4 distribution in lipid raft-enriched fractions. Immunoblotting analysis of membranes enriched in lipid rafts (fractions 1 to 6) and depleted of lipid rafts (fractions 7 to 10) in mock-, CXCL12-, SgG2- or SgG2:CXCL12-stimulated Jurkat cells. Cells were incubated with 15 nM CXCL12, 1.5 μM SgG2 or the complex CXCL12:SgG2 at 1:100 molar ratio (15 nM and 1.5 μM, respectively) for 15 min and then cell membranes were lysed in Triton X-100 and ultracentrifuged in a sucrose gradient. CXCR4 was analysed in the different membrane fractions along with the lipid raft marker GM1, detected by dot blot using HRP-conjugated cholera toxin. The protein LCK was also analysed as an additional marker for lipid raft-enriched membranes. Full blots are shown inSupplementary Fig. 5c. The experiment was performed twice with similar results. Molecular masses are indicated in kDa. Figure 3: SgG2 promotes clustering of lipid rafts and incorporation of CXCR4 to these microdomains. ( a ) Quantitative analysis of lipid rafts and CXCR4 co-localization. Jurkat T cells were transduced with the fluorescent lipid raft marker Lck 10 mCherry (in red), incubated with CXCL12 alone or in combination with SgG2 or PRV–SgG, and stained for endogenous CXCR4 (shown in green). Representative images from two independent assays are shown. The intensity correlation analysis (ICA) method was utilized to quantify co-localization of the fluorescent signals. As a result, two coefficients were calculated: Pearson’s coefficient (PC), which varies from −1 (perfect inverse correlation) to +1 (perfect positive correlation), and intensity correlation quotient (ICQ), which provides an overall index of whether the intensities are associated in a dependent or segregated manner (−0.5≤ICQ≤+0.5). Bar plots show PC and ICQ coefficient values obtained from 14 to 20 cells for a region of interest (ROI) corresponding to the entire plasma membrane. SgG2-induced focal clustering of lipid rafts and CXCR4 incorporation into these domains following cholesterol extraction with MβCD is also shown (lower row). BF, bright field. Scale bar, 2 μm. Data show mean±s.d. Two-tailed unpaired t -test, * P <0.05, ** P <0.01 ( b ) Analysis of CXCR4 distribution in lipid raft-enriched fractions. Immunoblotting analysis of membranes enriched in lipid rafts (fractions 1 to 6) and depleted of lipid rafts (fractions 7 to 10) in mock-, CXCL12-, SgG2- or SgG2:CXCL12-stimulated Jurkat cells. Cells were incubated with 15 nM CXCL12, 1.5 μM SgG2 or the complex CXCL12:SgG2 at 1:100 molar ratio (15 nM and 1.5 μM, respectively) for 15 min and then cell membranes were lysed in Triton X-100 and ultracentrifuged in a sucrose gradient. CXCR4 was analysed in the different membrane fractions along with the lipid raft marker GM1, detected by dot blot using HRP-conjugated cholera toxin. The protein LCK was also analysed as an additional marker for lipid raft-enriched membranes. Full blots are shown in Supplementary Fig. 5c . The experiment was performed twice with similar results. Molecular masses are indicated in kDa. Full size image Upon CXCL12 stimulation, the cell polarizes and GM3-enriched gangliosides are found at the leading edge, whereas GM1 gangliosides and adhesion molecules localize at the uropod [15] . CXCL12 stimulation of primary monocytes drove the accumulation of CXCR4 into GM3 rafts, as described [25] ( Fig. 4a ). Interestingly, SgG2 ( Fig. 4a ) and, to a lesser extent, SgG1 ( Supplementary Fig. 3b,c ) significantly increased the incorporation of CXCR4 into GM3 rafts in comparison with mock-treated cells. Contrary to SgG1 and SgG2, PRV–SgG blocked chemokine-promoted relocalization of CXCR4 to GM3-enriched areas in favour of a higher incorporation into GM1 rafts ( Fig. 4b ). In addition, although both GM1 and GM3 were upregulated in the presence of SgG2 ( Supplementary Fig. 4a,b ), CXCR4 was specifically redirected to clusters of GM3-enriched rafts ( Fig. 4 and Supplementary Fig. 4c,d ). 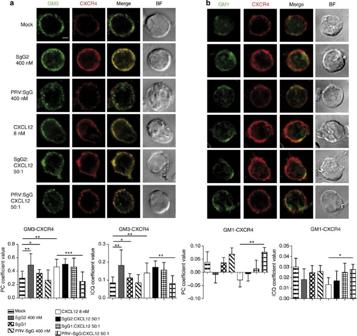Figure 4: HSV–SgG increases the localization of CXCR4 in GM3 rafts in primary human monocytes. Analysis of endogenous CXCR4 co-localization with GM3 and GM1 lipid rafts in freshly isolated monocytes. Cells were stimulated for 5 min at 37 °C as indicated, and then fixed and stained for (a) CXCR4 and GM3 rafts using specific antibodies or for (b) CXCR4 and GM1 lipid rafts using specific antibodies and FITC-conjugated cholera toxin B. Representative images are shown. Scale bar, 2 μm. Plots below the panels show the PC and ICQ values (mean±s.d.) obtained for the quantification of co-localization between CXCR4-GM3 and CXCR4-GM1 in 10 and 25 monocytes, respectively. The assay shown is representative of two independent assays. Two-tailed unpairedt-test was performed *P<0.05, **P<0.01, ***P<0.001. Figure 4: HSV–SgG increases the localization of CXCR4 in GM3 rafts in primary human monocytes. Analysis of endogenous CXCR4 co-localization with GM3 and GM1 lipid rafts in freshly isolated monocytes. Cells were stimulated for 5 min at 37 °C as indicated, and then fixed and stained for ( a ) CXCR4 and GM3 rafts using specific antibodies or for ( b ) CXCR4 and GM1 lipid rafts using specific antibodies and FITC-conjugated cholera toxin B. Representative images are shown. Scale bar, 2 μm. Plots below the panels show the PC and ICQ values (mean±s.d.) obtained for the quantification of co-localization between CXCR4-GM3 and CXCR4-GM1 in 10 and 25 monocytes, respectively. The assay shown is representative of two independent assays. Two-tailed unpaired t -test was performed * P <0.05, ** P <0.01, *** P <0.001. Full size image SgG2 modifies CXCR4 interaction with intracellular molecules Following CXCL12 stimulation, CXCR4 is phosphorylated at its cytosolic C-tail by GPCR-kinases (GRKs). This event determines the recruitment of β-arrestins to the cytoplasmic domain blocking further G-protein activation, desensitizing CXCR4 and regulating various trafficking events [12] , [26] . We analysed the phosphorylation status of the receptor in the presence of SgG2 using a phospho-specific antibody directed against phospho-serine 330 (pSer330), (ref. 26 ). SgG2 reduced the phosphorylation level of the steady-state receptor and inhibited chemokine-mediated phosphorylation ( Fig. 5a ). 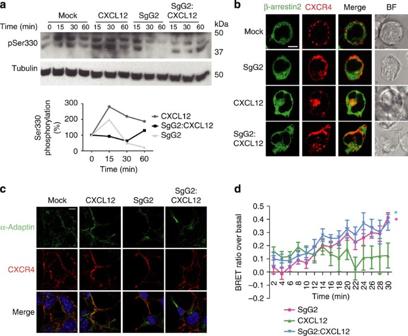Figure 5: Effect of SgG2 on the phosphorylation status of CXCR4 and its interaction with signalling molecules. (a) Western blot showing the phosphorylation of Ser330 residue (pSer330) on stimulation with CXCL12, SgG2 or SgG2:CXCL12. Blots were stripped and incubated with an anti-tubulin antibody as a loading control. Molecular masses in kDa are indicated. The graph below depicts the results obtained after performing densitometric analysis of the blots. The densities obtained from each lane were normalized to the loading control and later to the mock sample. One assay out of two is shown. Full blot is shown inSupplementary Fig. 5d. (b) Visualization of CXCR4 and β-arrestin-2 interaction. Selected frames from time-lapse videos showing the redistribution of GFP-β-arrestin-2 and RFP-CXCR4 in Jurkat T cells following 15 min stimulation. Scale bar, 2 μm. (c) Immunofluorescence showing the interaction of CXCR4 with the clathrin-dependent endocytic machinery. Flag-CXCR4-expressing HEK-293T cells were stimulated for 5 min with CXCL12, SgG2 or SgG2:CXCL12. Cells were fixed, permeabilized and stained for CXCR4 and α-adaptin. Scale bar, 10 μm. (d) BRET2ratio over the value obtained for mock-treated cells expressing CXCR4-GFP2and CXCR4-luc. HEK-293T cells were stimulated with 15 nM CXCL12, 1.5 μM SgG2 or the complex SgG2:CXCL12 at a 100:1 molar ratio. Three independent assays performed in triplicates are represented. One-tailed unpairedt-test, *P<0.05. Figure 5: Effect of SgG2 on the phosphorylation status of CXCR4 and its interaction with signalling molecules. ( a ) Western blot showing the phosphorylation of Ser330 residue (pSer330) on stimulation with CXCL12, SgG2 or SgG2:CXCL12. Blots were stripped and incubated with an anti-tubulin antibody as a loading control. Molecular masses in kDa are indicated. The graph below depicts the results obtained after performing densitometric analysis of the blots. The densities obtained from each lane were normalized to the loading control and later to the mock sample. One assay out of two is shown. Full blot is shown in Supplementary Fig. 5d . ( b ) Visualization of CXCR4 and β-arrestin-2 interaction. Selected frames from time-lapse videos showing the redistribution of GFP-β-arrestin-2 and RFP-CXCR4 in Jurkat T cells following 15 min stimulation. Scale bar, 2 μm. ( c ) Immunofluorescence showing the interaction of CXCR4 with the clathrin-dependent endocytic machinery. Flag-CXCR4-expressing HEK-293T cells were stimulated for 5 min with CXCL12, SgG2 or SgG2:CXCL12. Cells were fixed, permeabilized and stained for CXCR4 and α-adaptin. Scale bar, 10 μm. ( d ) BRET 2 ratio over the value obtained for mock-treated cells expressing CXCR4-GFP 2 and CXCR4-luc. HEK-293T cells were stimulated with 15 nM CXCL12, 1.5 μM SgG2 or the complex SgG2:CXCL12 at a 100:1 molar ratio. Three independent assays performed in triplicates are represented. One-tailed unpaired t -test, * P <0.05. Full size image We next analysed the distribution of β-arrestin-2 and CXCR4 in Jurkat cells. SgG2 reduced the intracellular accumulation of the receptor into β-arrestin-2-positive vesicles ( Fig. 5b ). The diminished interaction with β-arrestin-2 correlated with a reduced co-localization between CXCL12-activated CXCR4 and α-adaptin, suggesting an impaired interaction of the receptor with the clathrin-dependent endocytic machinery ( Fig. 5c ). This observation was consistent with the increased presence of CXCR4 at the surface of SgG2-stimulated cells. Furthermore, by performing bioluminescence resonance energy transfer (BRET) assays using GFP- and luciferase-tagged CXCR4, we observed that SgG2 triggered specific time-dependent conformational rearrangements within CXCR4 homodimers, different to those induced by CXCL12 alone ( Fig. 5d ). SgG2 function depends on lipid raft integrity We next measured the migration of freshly isolated human monocytes and MM-1 cells in the presence of chemical inhibitors of clathrin-coated pits (CCP) formation (chlorpromazine) or lipid raft disrupting or sequestering reagents (filipin, nystatin and MβCD). SgG2 displaced the chemotactic curve towards lower concentrations of the chemokine, whereas PRV:SgG inhibited chemotaxis ( Fig. 6a ), as previously shown [5] . Perturbation of lipid raft formation by filipin slightly affected migration towards CXCL12, but it completely abrogated SgG2-mediated enhancement ( Fig. 6b ). On the contrary, the inhibition of CCP formation did not significantly abolish SgG2-mediated potentiation of monocyte chemotaxis ( Fig. 6c ). The doses of chlorpromazine used in the migration assays were proven to be functional, as indicated by the blockade of the transferrin-induced CD71 endocytosis ( Supplementary Fig. 5e ). In addition, disruption of lipid raft integrity by distinct compounds (nystatin and MβCD) inhibited SgG2-induced increase in CXCL12-mediated migration ( Fig. 6d,e ). To further determine the signalling pathways involved in chemotaxis potentiation, we utilized Ly294002, a compound blocking phosphoinositide 3-kinase (PI3K) function and PP2, an inhibitor of Src-kinases. Both abrogated SgG2-induced increase of chemotaxis ( Fig. 6f,g ). 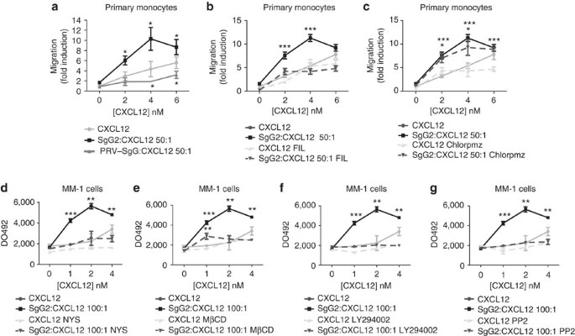Figure 6: HSV SgG2-mediated enhancement of chemokine function depends on lipid raft integrity but it does not require clathrin-coated pit formation. (a–c) Analysis of human primary monocyte migration by transwell. (a) Migration towards a range of CXCL12 concentrations alone or in the presence of a 50:1 molar ratio of SgG2 or PRV–SgG. (b) Chemotaxis in the presence of filipin (FIL) or (c) chlorpromazine (chlorpmz). The induction of migration depicted is from one assay performed in triplicate (a) or two assays performed in triplicate (b,c). (d–g) Transwell experiments showing MM-1 cell migration towards a range of low concentrations of CXCL12 or SgG2:CXCL12 in a 100:1 molar ratio in the absence or presence of different chemical inhibitors. (d) Impact of the perturbation of lipid raft assembly by nystatin (NYS) and (e) MβCD on the function exerted by SgG2. (f) Migration in the presence of the selective inhibitor of Ly294002, an inhibitor of PI3K activity or (g) PP2, an inhibitor of Src Kinase. Plots show one representative assay performed in triplicate out of at least three independent experiments. Error bars represent s.d. Two-tailed unpairedt-test, *P<0.05, **P<0.01,***P<0.001. Figure 6: HSV SgG2-mediated enhancement of chemokine function depends on lipid raft integrity but it does not require clathrin-coated pit formation. ( a – c ) Analysis of human primary monocyte migration by transwell. ( a ) Migration towards a range of CXCL12 concentrations alone or in the presence of a 50:1 molar ratio of SgG2 or PRV–SgG. ( b ) Chemotaxis in the presence of filipin (FIL) or ( c ) chlorpromazine (chlorpmz). The induction of migration depicted is from one assay performed in triplicate ( a ) or two assays performed in triplicate ( b , c ). ( d – g ) Transwell experiments showing MM-1 cell migration towards a range of low concentrations of CXCL12 or SgG2:CXCL12 in a 100:1 molar ratio in the absence or presence of different chemical inhibitors. ( d ) Impact of the perturbation of lipid raft assembly by nystatin (NYS) and ( e ) MβCD on the function exerted by SgG2. ( f ) Migration in the presence of the selective inhibitor of Ly294002, an inhibitor of PI3K activity or ( g ) PP2, an inhibitor of Src Kinase. Plots show one representative assay performed in triplicate out of at least three independent experiments. Error bars represent s.d. Two-tailed unpaired t -test, * P <0.05, ** P <0.01,*** P <0.001. Full size image gG2 increases CXCR4 nanoclusters at the cell surface To assess whether SgG2-mediated increase in cell responsiveness to the chemokine was related to changes in the oligomerization state of CXCR4, as well as to address the effect on the receptor by means of a higher resolution technique, we prepared surface replicas by label-fracture of Jurkat T cells [27] , [28] , which were analysed by electron microscopy ( Fig. 7 ). We observed a significant increase in the amount of small clusters of CXCR4 (oligomers formed by ≤6 gold particles) at the surface of T cells stimulated with SgG2, in comparison with mock- and CXC12-treated cells ( Fig. 7 ). The percentage of clusters containing 2, 3 and 4–9 gold particles, respective to the total number of particles in each case, was also increased in SgG2 and SgG2:CXCL12-stimulated cells ( Fig. 7e , left inset). In parallel, a reduction in the percentage of CXCR4 monomers in cells treated with SgG2 was observed compared with the mock-treated cells ( Fig. 7e , left inset). Moreover, consistent with our previous results, we observed a significant enhancement in the total number of gold particles in SgG2-treated cells ( Fig. 7e , right inset). Representative whole-cell replica images corresponding to CXCL12- and SgG2:CXCL12-stimulated cells are shown in Supplementary Figs 6 and 7 . Similar results were obtained for HEK-293T cells stably expressing CXCR4 ( Supplementary Fig. 8 ). 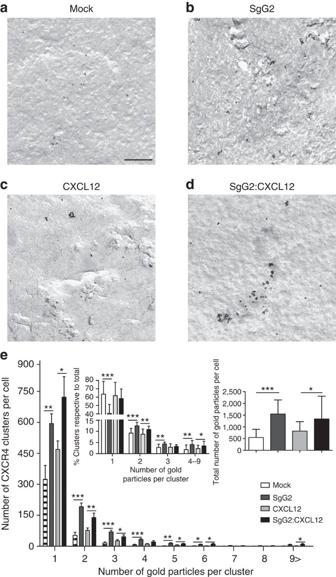Figure 7: Effect of SgG2 on the nanoclustering of CXCR4 at the cell surface of T cells. The number and size of clusters present in the replicas of individual cells was determined by electron microscopy. Selected small field images ( × 10.000) showing the distribution of gold particles in cell surface replicas of (a) mock-treated cells, and (b) 1.5 μM SgG2-, (c) 15 nM CXCL12- or (d) 100:1 molar ratio SgG2:CXCL12-stimulated cells. Scale bar, 200 nm. (e) Quantification of gold particle distribution for each experimental condition (mean±s.e.m.). Data from eight mock-treated cells (4,380 gold particles), 17 SgG2-stimulated cells (26,291), 18 CXCL12-stimulated cells (14,476) and 17 SgG2:CXCL12-stimulated cells (22,683) from two independent assays are represented. (e, left inset) The plot shows the percentage of clusters of the indicated sizes respective to the total number of gold particles found in each experimental condition (mean±s.d.). (e, right inset) Representation of the average total number of gold particles per cell (mean±s.d.). One-tailed unpairedt-test, *P<0.05, **P<0.01, ***P<0.001. Figure 7: Effect of SgG2 on the nanoclustering of CXCR4 at the cell surface of T cells. The number and size of clusters present in the replicas of individual cells was determined by electron microscopy. Selected small field images ( × 10.000) showing the distribution of gold particles in cell surface replicas of ( a ) mock-treated cells, and ( b ) 1.5 μM SgG2-, ( c ) 15 nM CXCL12- or ( d ) 100:1 molar ratio SgG2:CXCL12-stimulated cells. Scale bar, 200 nm. ( e ) Quantification of gold particle distribution for each experimental condition (mean±s.e.m.). Data from eight mock-treated cells (4,380 gold particles), 17 SgG2-stimulated cells (26,291), 18 CXCL12-stimulated cells (14,476) and 17 SgG2:CXCL12-stimulated cells (22,683) from two independent assays are represented. ( e , left inset) The plot shows the percentage of clusters of the indicated sizes respective to the total number of gold particles found in each experimental condition (mean±s.d.). ( e , right inset) Representation of the average total number of gold particles per cell (mean±s.d.). One-tailed unpaired t -test, * P <0.05, ** P <0.01, *** P <0.001. Full size image Dysregulation of the chemokine network affects the onset of viral infections and the development of immunopathologies. Here, we have addressed the molecular basis regulating the first example of chemokine potentiation by a viral protein [5] . Our results show that HSV–SgG interaction with the cell leads to the enrichment of oligomeric chemokine receptor complexes and their sustainment at the cell surface. Although a correlation between an augmented presence of CXCR4 at the surface and an improved chemotactic response has been previously reported [29] , [30] , our studies constitute the first description of a pathogen-encoded protein that modifies GPCR trafficking and plasma membrane architecture as a novel immunomodulatory strategy. SgG2 interacts with GAGs and induces lipid raft clustering, promoting the incorporation of CXCR4 into these specific microdomains and altering receptor trafficking. GPCRs have seven transmembrane domains and therefore are highly dependent on structural and functional regulation by lipids. In fact, cholesterol modulates GPCR function either by direct interaction with the receptor and/or by altering the plasma membrane environment where the receptor is embedded, a regulation that seems to be receptor specific [31] , [32] . Thus, the fate of different types of receptors following SgG2 stimulation could depend on the affinity and degree of dependency of each receptor for cholesterol. In accordance with this hypothesis, SgG2 did not significantly modify the internalization of CD71, a receptor with a very low tendency to interact with cholesterol and that is commonly found outside lipid rafts [33] , whereas it modified the trafficking of all GPCRs assayed (CXCR4, CXCR5 and CCR2). Interestingly, contrary to what we observed for CXCR4 and CXCR5, whose cognate chemokines interact with SgG, SgG2 did not potentiate CCL2-mediated migration [5] , in spite of the increase on surface CCR2 upon SgG2 stimulation. These observations indicate that, besides the stabilization of the chemokine receptor at the surface, the chemokine needs to be presented to its receptor as a complex with the viral protein, further supporting our hypothesis that SgG2 mimics the role of GAGs presenting chemokines to their receptors [5] ( Fig. 8 ). Alternatively, chemokine binding by SgG2 may increase the local chemokine concentration in the proximity of the chemokine receptor. 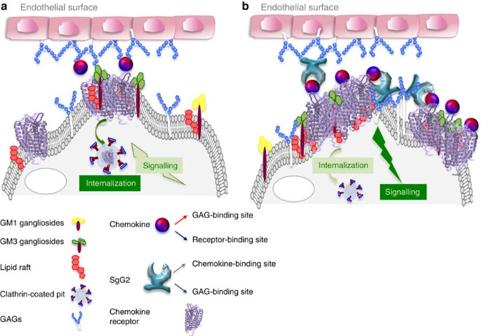Figure 8: Proposed model for SgG2 mechanism of action. (a) Chemokines are retained at the cell surfaces through their interaction with GAGs, which modify the quaternary structure of the chemokine improving the presentation to its receptor. (b) SgG2 is secreted to the extracellular environment where it binds chemokines through the GAG-binding domain of the chemokine, leaving the receptor-binding site available to interact with the GPCR. SgG2 associates to the cell through an interaction with GAG-containing proteins, triggering patching of lipid raft-associated molecules and an increased clusterization of chemokine receptors into these microdomains. In this scenario, SgG2 increases the local concentration of the chemokine, acting as a viral GAG that improves chemokine presentation to its GPCR. The receptors included in a particular microenvironment of the plasma membrane may couple more efficiently to specific signalling partners, leading to a delayed internalization and an increased signalling in response to SgG2:chemokine stimulation. The combination of receptor relocalization to particular microdomains on the cell surface together with the presentation of the chemokine as a complex with SgG2 provides a molecular explanation for the enhancement of chemokine functions. Figure 8: Proposed model for SgG2 mechanism of action. ( a ) Chemokines are retained at the cell surfaces through their interaction with GAGs, which modify the quaternary structure of the chemokine improving the presentation to its receptor. ( b ) SgG2 is secreted to the extracellular environment where it binds chemokines through the GAG-binding domain of the chemokine, leaving the receptor-binding site available to interact with the GPCR. SgG2 associates to the cell through an interaction with GAG-containing proteins, triggering patching of lipid raft-associated molecules and an increased clusterization of chemokine receptors into these microdomains. In this scenario, SgG2 increases the local concentration of the chemokine, acting as a viral GAG that improves chemokine presentation to its GPCR. The receptors included in a particular microenvironment of the plasma membrane may couple more efficiently to specific signalling partners, leading to a delayed internalization and an increased signalling in response to SgG2:chemokine stimulation. The combination of receptor relocalization to particular microdomains on the cell surface together with the presentation of the chemokine as a complex with SgG2 provides a molecular explanation for the enhancement of chemokine functions. Full size image Our results support previous studies suggesting that CXCR4 incorporation into lipid rafts improves the signalling properties of the receptor [30] , [34] . Furthermore, SgG induced a specific association of CXCR4 with GM3-enriched rafts, a subtype of lipid rafts found at the leading edge of migrating leukocytes, whereas it decreased its incorporation into GM1 or uropod-rafts. SgG2-induced redistribution of CXCR4 may improve receptor coupling to specific pathways, making the cell more prone to sense threshold concentrations of chemokines that would otherwise be insufficient to trigger functional responses. This effect may account in part for the faster and more directional movement observed in primary monocytes [5] . In contrast, gG from PRV, a related protein that inhibits chemokine activity [21] , prevents the relocalization of CXCR4 to GM3-containing rafts. Alterations in receptor distribution at the membrane may modulate its initial interaction with signalling molecules [12] , [35] . A higher interaction with cholesterol may regulate different aspects of CXCR4 function, either by promoting more active conformations of the receptor or by creating a platform for the association with a specific set of signalling proteins [30] , [32] , [36] . We have shown that SgG2-induced redistribution of receptors drives a conformational rearrangement in CXCR4 dimers distinct to that caused by CXCL12. We propose that such rearrangements are transmitted to the cytosolic domain of the GPCR, leading to a differential recruitment of signalling molecules. In line with our hypothesis, it has been previously shown that CXCR4 changes its G-protein-coupling specificity when the receptor relocates to the T-cell immune synapse, a structure characterized by lipid raft clustering [37] . The alterations we have observed in the phosphorylation pattern of CXCR4 C-tail could explain the diminished recruitment of β-arrestin and the differential interaction with the canonical clathrin-dependent endocytic machinery [12] , [35] , which would ultimately account for the overall alterations in trafficking and the increased functionality of surface chemokine receptors on exposure to SgG2. Our results provide additional evidence for the observation that functional association of CXCR4 with Src- and PI3K-signalling routes in the lipid raft microenvironment leads to an increased sensitization to chemokines [34] , [38] , [39] . Furthermore, the observation that CXCR4 is displaced from CCPs and the increased association of the complex CXCL12/CXCR4 with lipid raft markers could indicate that chemokine receptors act as ‘lipid-raft-biased’ receptors in the presence of the viral protein. Although the oligomerization of some chemokines has been proven important for receptor activation [40] , [41] , whether chemokine receptors are active as monomers, dimers or higher order oligomers remains poorly understood [42] , [43] . Growing evidence suggests that non-stimulated receptors co-exist in an equilibrium of inactive and active conformations, which shifts towards specific receptor conformations depending on the ligand triggering the response. It is well accepted that CXCR4 is able to oligomerize in the absence of chemokine [44] , [45] , [46] . However, to our knowledge, there are no clear reports showing the correlation between CXCR4 aggregation state and its biological activity. We have clearly demonstrated that SgG2 enhances the functionality of the CXCR4/CXCL12 pair using signalling and chemotaxis experiments as readout for cell activation. Interestingly, we found that such enhanced activation associated with a significant increase in the amount of receptor nanoclusters and their relative percentage at the surface of SgG2-stimulated cells. We propose that the reorganization of the receptor in nanoclusters located at particular subdomains of the plasma membrane predisposes the receptor to establish a more efficient interaction with signalling partners, improving cell responsiveness to suboptimal concentrations of the chemokine. Proteoglycans (PGs) are GAG-rich signalling co-receptors that serve as scaffolds for multiple signalling complexes, playing key roles during processes such as adhesion, cell activation or protein polarization at the leading edge of migrating cells [47] . Ligand binding induces PG clusterization within lipid rafts, a process that has been related to a PG-dependent route of endocytosis distinct to that mediated by clathrin [48] , [49] . A reasonable explanation for the phenomena described in this report is that SgG binds PGs through their extracellular GAGs, leading to PGs patching into cholesterol-rich domains, where GPCR inclusion is enhanced. In that scenario, SgG may mimic the function of GAGs, modifying the quaternary structure of the chemokine presenting it in an optimal spatial conformation to SgG2-induced CXCR4 oligomers and increasing the effective activity of CXCL12. SgG2 could also increase the concentration of the chemoattractant in the local environment of the receptor thereby increasing the avidity for receptor binding. During HSV-2 infection, SgG could immediately bind to the surface of the infected cell, or neighbouring cells, modifying the interaction of GPCRs with chemokines produced in the infected mucosa and enhancing the biological activity of chemokines. Although the function of SgG in vivo requires further investigation, we can hypothesize several scenarios where SgG activity could promote HSV infection. (i) Cell activation could favour viral replication; for example, downstream effectors or GPCR signalling, such as MAPKs, are required for efficient HSV replication [50] . (ii) We have shown that SgG enhances the activity of non-proinflammatory chemokines [5] , and SgG could selectively modify the population of infiltrating leukocytes, which, in turn, could be infected increasing viral loads and spread, or modulate the immune response facilitating viral immune evasion. (iii) Membrane remodelling and receptor trafficking modulation by SgG could serve as a mechanism to increase the availability of HSV entry receptors. In addition, the dysregulation of the chemokine receptor trafficking by HSV, in particular that of CXCR4, may contribute in part to the enhanced susceptibility to HIV infection reported in co-infected individuals [51] . (iv) Finally, the well-documented increased risk of HIV-1 infection and transmission due to HSV-2 infection [52] may be partially due to the activation and enhancement of T-cell migration by HSV-2 (refs 53 , 54 ). Whether HSV-2 gG plays a role in these scenarios requires further investigation. Membrane trafficking controls many complex and diverse biological responses, including those triggered by chemokines. Since chemokines coordinate functions that go beyond the immune response, the modulation of chemokine receptor trafficking suggests a role for gG at other stages of HSV infection, such as the initial colonization of the nervous system, where chemokines including CXCL12 have an important regulatory function. In fact, we have found that SgG2 modifies the trafficking and signalling of the neutrophic growth factor-receptor TrkA, leading to an increase in axonal growth [55] . This work provides a molecular explanation for HSV gG modulation of chemokine activity. The insights presented here shed light into basic concepts of the chemokine network biology, receptor trafficking and HSV immune modulation. To our knowledge, HSV gG is the first vCKBP encoded by a human pathogen that regulates cell receptor trafficking and oligomerization through the modification of lipid raft architecture. Cells and plasmids Jurkat (human, peripheral blood, leukemia, T cell) and MonoMac-1 (MM-1, human, monocyte-like) cells were grown in RPMI 1640 (Sigma) containing 10% fetal bovine serum (FBS) (R-10 medium). m300-19-hCXCR5 (stably transfected with hCXCR5) were a gift of Dr Bernhard Moser (Cardiff University) and were grown in R-10 medium supplemented with β-mercaptoethanol (5 × 10 −5 M), sodium pyruvate (1%) and puromycin (1.5 μg ml −1 ). HEK-293T, MDCK and Vero cells were grown in Dulbecco’s Modified Eagle’s medium (DMEM) containing 10% FBS. CHO-K1 and CHO-618 cells were grown in DMEM-F12 1:1 medium containing 10% FBS. All mammalian cell lines were cultured at 37 °C, 5% CO 2 in a humidified incubator. The ACP-CXCR4 HEK-293T cells and the Lck 10 mCherry expressing HEK-293T and MDCK cell lines were generated by lentiviral transduction, as previously described [56] . All the cell lines were acquired from the ATCC unless indicated. Chemokines Chemokines were obtained from Peprotech (London). CXCL12α-biotin, kindly provided by I. Clark Lewis, was conjugated with Quantum Dots (Qdots)–streptavidin (Invitrogen) at a ratio 4:1 (CXCL12-biotin/QD605, mol per mol) for 15 min at room temperature (RT) immediately before the experiments. Generation and purification of recombinant proteins Recombinant proteins were generated using the recombinant baculovirus expression system followed by protein purification by affinity chromatography [5] , and the purified proteins were dialysed against HEPES buffer using a Vivaspin500 device (VivaScience). The SgG1, SgG2 and PRV–SgG constructs used in this study have been previously described [5] , [21] . Lentiviral transduction, transfection and electroporation of cell lines Supernatants used in transduction experiments were produced transfecting packaging HEK-293T cells with pALPS-CXCR4 or pALPS-Lck 10 mCherry, psPAX2 and pMD2-G plasmids, as described [56] . Jurkat cells were incubated with the supernatants during 72–96 h in the presence of 4 μg ml −1 polybrene (Sigma). Transfection of mammalian cells was carried out using Fugene HD reagent (Promega). Jurkat cells (20–30 × 10 6 ) in Opti-MEM medium (Gibco) were mixed with 10–30 μg DNA, electroporated in an EasyjecT apparatus (Eurogentec, Belgium), and grown overnight in R-10 medium. Isolation of human monocytes Monocytes were prepared from buffy coats obtained from the local donor bank (‘Servizio Trasfusion, Svizzera Italiana’, Lugano, Switzerland) with oral consent from the donors according to Swiss regulations. The use of buffy coats was approved by the institutional review board ‘Comitato Etico Cantonale, Bellinzona, Switzerland’. Monocytes were isolated using the Monocyte Isolation kit II (MACS Miltenyi Biotec), following manufacturer’s instructions. In brief, peripheral blood mononuclear cells were isolated from heparinized blood by Ficoll (Lymphoprep) gradient centrifugation and incubated with FcR blocking reagent. Highly enriched unlabelled monocytes were obtained by negative selection. Analysis of protein binding to cells Cells were incubated on ice for 30 min with purified proteins or virus-free supernatants from HSV-2-infected cells. Protein binding was assessed by flow cytometry using an in-house generated rabbit polyclonal antibody against SgG1, an anti-gG2 antibody (20 μg ml −1 ) (Austral Biologicals) or an anti-His tag antibody (10 μg ml −1 ) (QIAGEN) to detect vaccinia virus B18 and ectromelia virus semaphorin (sema) proteins, followed by Alexa Fluor 488 donkey anti-mouse IgG secondary antibody (Invitrogen) used at 4 μg ml −1 . The anti-SgG1 antibody was generated by injecting purified recombinant SgG1 into one rabbit. To analyse the binding by immunofluorescence, the cells were washed after incubation with the viral proteins, fixed with 4% paraformaldehyde (PFA) and subsequently stained using a monoclonal anti-SgG1 antibody (LP-10, kindly provided by Helena Browne, Cambridge University, UK), an anti-SgG2 polyclonal antibody (Austral Biologicals), an anti-His tag antibody (QIAGEN) to detect B18 and sema, and a polyclonal antibody to detect CXCR4 (Abcam) in the case of monocytes, which were incubated for 15 min at 4 °C or 37 °C with 400 ng of SgG2 alone or in combination with CXCL12. SPR assays for SgG-heparin binding and GAG competition Kinetic studies were perfomed injecting different concentrations of SgG2 over a streptavidin sensor chip (BIAcore) with immobilized biotinylated heparin [17] . Bulk refractive index changes were removed and curves were globally fitted using a 1:1 mass transport binding model. For competition assays, SgG2 (100 nM) was incubated with different concentrations of soluble GAGs (Sigma), including heparin, heparan sulfate, chondroitin sulfate A and chondroitin sulfate B for 10 min. The mixture was injected over a heparin-SA sensor chip at a 10 μl min −1 flow rate, and the response at equilibrium was recorded. All the assays were run in HBS-EP buffer (10 mM Hepes, 150 mM NaCl, 3 mM EDTA, 0.005% (vol/vol) surfactant P20, pH 7.4). Heparin–agarose-based pull-down assay Different concentrations of SgG2 were incubated for 1 h at RT with heparin–agarose beads (Sigma) in binding buffer (0.2% bovine serum albumin (BSA) in phosphate-bufffered saline (PBS)). The beads were washed three times with PBS and bound viral proteins were eluted with SDS–polyacrylamide gel electrophoresis (SDS–PAGE) loading buffer, and then subjected to SDS–PAGE and detected by immunoblotting. ACP labelling reaction CXCR4 was engineered with a tag at the amino (N) terminus derived from the ACP and the labelling reaction was performed as described [22] . Briefly, the cells were washed with PBS containing calcium and magnesium and incubated for 15 min at RT with 5 μM CoA-Atto dye in the presence of the enzyme (1 μM PPTase). The cells were washed to remove excess of dye and immediately processed for time-lapse or immunofluorescence. Since the reagents used are non-cell permeable, this methodology enables the specific labelling of surface CXCR4 (ref. 22 ). Receptor internalization assays The amount of surface CXCR4 was analysed by flow cytometry in MM-1 cells, Jurkat cells and primary monocytes. Cells were mock treated or incubated with 1.5 μM SgG or PRV–SgG, 15 nM CXCL12 or the complex vCKBP:CXCL12 at a 50:1 or 100:1 molar ratio for different time points. After incubation at 37 °C with the different stimuli, cells were kept at 4 °C at all times, and CXCR4 remaining at the surface was detected by flow cytometry using a PE-conjugated anti-CXCR4 antibody (R&D Systems). m300-19-hCXCR5 cells were incubated with 15 nM CXCL13, 1.5 μM SgG2 or SgG2:CXCL13 at a 100:1 molar ratio for 15 min at 37 °C. The cells were incubated with a PE-conjugated anti-CXCR5 antibody (R&D Systems) at 4 °C, and then surface receptor was analysed by flow cytometry. Similarly, for CCR2 analysis, MM-1 cells were incubated with 5 nM CCL2, 500 nM SgG2 or a combination of SgG2 and CCL2 at a 1:100 nM ratio for 15 min and the level of surface CCR2 was analysed by flow cytometry using an APC-conjugated anti-CCR2 antibody (R&D Systems). For CD71 internalization studies, MM-1 cells were serum starved for 1 h before the assay, and then stimulated with 1 mg ml −1 transferrin (Sigma), 1.5 μM SgG2 or both. The cells were incubated with anti-CD71 (BD Pharmingen) and anti-mouse Alexa488-conjugated antibody (Invitrogen) and receptor levels at the surface were analysed by flow cytometry. Data were collected on a FACSCalibur (Becton Dickinson) and analysed using FlowJo 7.2.2 software (Treestar). The values obtained for each experimental condition were represented as a percentage of the values corresponding to mock-treated cells, which were assigned 100%. Typically, 10 5 cells were stained using 2 μl of the indicated antibodies per reaction. Analysis of CXCR4 incorporation into Lck 10 mCherry rafts Jurkat cells transduced with a lentiviral vector expressing the fluorescent lipid raft marker Lck 10 mCherry were stimulated for 30 min with 8 nM CXCL12, 800 nM SgG2 or PRV–SgG or the vCKBP:CXCL12 complex at a 100:1 molar ratio and then fixed with 4% ice-cold PFA. Subsequently, a polyclonal antibody (Abcam) was used (10 μg ml −1 ) to detect endogenous CXCR4. Analysis of lipid raft clustering Jurkat cells transduced with the fluorescent lipid raft marker Lck 10 mCherry were stained with Vybrant DiO plasma membrane marker (Molecular Probes) following manufacturer’s instructions. Afterwards, the cells were incubated for 30 min at 37 °C with 8 nM CXCL12, 800 nM SgG2 or PRV–SgG or the vCBKPs:CXCL12 at a 100:1 molar ratio and subsequently fixed with 4% PFA. Pseudocoloured images showing Lck 10 mCherry clustering were obtained using Image J software. To investigate GM3 lipid raft clustering, Jurkat cells were stained using the plasma membrane marker Vybrant DiD (Molecular Probes) and stimulated for 15 min at 37 °C using 8 nM CXCL12, 800 nM SgG1, SgG2 or PRV–SgG or the vCKBP in combination with chemokine at a 100:1 molar ratio. The cells were fixed with 4% PFA and GM3 lipid rafts and CXCR4 were detected using a specific antibody against GM3 (ref. 25 ) and a polyclonal antibody recognizing the receptor (Abcam). A region of interest corresponding to the perimeter of the plasma membrane was selected to generate the qualitative intensity histograms. The area corresponding to GM1 and GM3 staining was analysed in primary monocytes. The cells were stimulated with SgG1, SgG2, PRV–SgG, CXCL12 or the vCKBPs:CXCL12 for 15 min at 37 °C, fixed with PFA and stained to detect GM3 and GM1. The images were subjected to background correction and threshold analysis to quantify the area corresponding to the different types of lipid raft staining using Image J software. CXCL12 immunofluorescence and receptor phosphorylation HEK-293T cells expressing ACP-tagged CXCR4 were ACP-labelled and subsequently mock treated or incubated with 8 nM CXCL12α-biotin/Qdots, 800 nM SgG2 or the complex SgG2:CXCL12α-biotin/Qdots at a 100:1 molar ratio for 30 min at 37 °C. Afterwards, the cells were recorded for 30 min at 37 °C. For the quantification of CXCL12 and CXCR4 co-localization, ACP-CXCR4 HEK-293T cells were ACP-labelled and treated with 8 nM CXCL12-biotin/Qdots alone or in the presence of 800 nM SgG2. The cells were fixed with PFA after 30 min of stimulation at 37 °C and chemokine/receptor co-localization was quantified using Image J software. To analyse the localization of CXCL12, ACP-CXCR4 HEK-293T cells were incubated during 45 min at 37 °C with 8 nM CXCL12-biotin/Qdots alone or in the presence of 800 nM SgG2. Subsequently, the cells were washed with an acidic buffer (glycine-HCl pH 3) for 30 s at 4 °C following fixation with PFA 4%. The area corresponding to the CXCL12 fluorescent signal was determined using Image J software. Binding of CXCL12α-biotin/Qdots to lipid rafts was analysed in MDCK cells stably expressing the Lck 10 mCherry marker. The cells were incubated with 8 nM CXCL12-biotin/Qdots, alone or in the presence of SgG2 (800 nM) for 30 min at 37 °C, and then fixed with 4% PFA. In both the experiments, images were acquired using a Leica TCS SP5 confocal laser microscope. For the analysis of CXCR4 and AP-2 co-localization, Flag-CXCR4-expressing HEK-293T cells were stimulated with CXCL12, SgG2 or SgG2:CXCL12 for 5 min at 37 °C, and immediately fixed and permeabilized with PBS containing 0,5% Triton X-100. Afterwards, the cells were stained using antibodies directed against the Flag tag (Sigma) and endogenous α-adaptin (BD Pharmingen). The images were acquired using a Leica TCS SP5 confocal laser microscope. Flag-CXCR4-expressing HEK-293T cells were serum starved and then stimulated with 8 nM CXCL12, 800 nM SgG2 or SgG2:CXCL12 at a 100:1 molar ratio (15–60 min). After stimulation, the cells were lysed using 2 × SDS-loading buffer and then centrifuged at 20,000 g for 15 min. Samples were not boiled to minimize receptor aggregation. Blots were incubated overnight in TBS-Tween buffer containing 0.25% gelatin with the phospho-specific antibody anti-pSer330. Membranes were stripped and probed with anti-tubulin as a loading control (Sigma). Isolation of lipid raft-enriched membrane fractions Jurkat cells were stimulated with 15 nM CXCL12, 1.5 μM SgG2, the complex SgG2:CXCL12 at a 100:1 molar ratio or mock treated for 15 min and then washed in HNEX buffer (25 mM Hepes, 5 mM EDTA, 150 mM NaCl). A total of 50 × 10 7 cells were used per condition. The cells were lysed in HNEX containing 0.5% Tritron X-100 and then overlaid with a sucrose gradient (0.2–0.9 M sucrose in HNEX). After centrifugation at 287,000 g in a SW41 rotor for 16 h, fractions were collected from top to bottom and proteins were precipitated by adding TCA. The pellets were washed and solubilized in Trizma buffer pH 9 (Sigma) by brief sonication in an ultrasound bath. Some of the fractions corresponding to lipid rafts were pooled, as indicated, and samples from all the fractions were analysed by western blot using specific antibodies against CXCR4 (Abcam) or LCK (kindly provided by M.A. Alonso, CBMSO, Spain). GM1 was detected by dot blot using HRP-conjugated cholera toxin (20 μg ml −1 ) (Sigma). Analysis of primary monocyte polarization Freshly isolated monocytes were adhered to coverslips coated with poly- D -lysine (Sigma) and the cells were mock treated or stimulated with 8 nM CXCL12, 800 nM SgG1, SgG2 or PRV–SgG or with the vCKBPs:CXCL12 complex at a 50:1 molar ratio for 5 min at 37 °C. After stimulation, the cells were PFA-fixed and stained using a polyclonal antibody against CXCR4 (Abcam) and an anti-GM3 antibody [25] or FITC-conjugated cholera toxin β-subunit (5 μg ml −1 ) (Sigma) to detect GM3 and GM1 lipid rafts, respectively. Chemotaxis assays Primary monocyte or MM-1 cell migration was analysed using 96-well ChemoTx plates (Neuro Probe) [5] . Cells were incubated with the chemical inhibitors for 30 min at 37 °C before the assay and the drugs were maintained during the migration assay. The inhibitors were used at the following concentrations: 7 mM MβCD (Sigma), 50 μg ml −1 filipin (Sigma), 1.5 μg ml −1 nystatin (Sigma), 2 μM chlorpromazine (Sigma), 10 μM Src kinase inhibitor PP2 (Sigma) and 35 μM PI3K inhibitor LY294002 (Calbiochem). The plates were incubated at 37 °C for 1 h (primary monocytes) or 2–3 h (MM-1 cells) and the number of migrated cells was determined by staining the cells in the lower chamber with 5 μl of CellTiter 96 aqueous one solution (Promega) in the case of MM-1 cells. Primary monocytes were counted with a light microscope. BRET assays BRET assays were performed as previously described with minor modifications [26] . Briefly, HEK-293T cells were transfected with the donor construct Rluc-CXCR4 (0.1 μg) and acceptor construct GFP 2 -CXCR4 (1 μg) using Fugene HD reagent (Promega) in 6-well plates and the total amount of DNA was adjusted to 2 μg with empty vector. The cells were detached 24 h later and seeded at 5 × 10 5 cells per well in 96-well white plates (Corning) pretreated with poly- D -lysine and poly- L -ornithine and cultured for an additional 24 h. The growing medium was replaced with PBS containing 0.1% (w/v) glucose for 1 h before the assay. The cells were treated with 1.5 μM SgG2, 15 nM CXCL12 or both at a 100:1 molar ratio before the addition of freshly prepared DeepBlueC (DBC, 5 μM). BRET readings were collected immediately after DBC addition, using a multidetector plate reader (Tecan Infinite F500). BRET signal was determined by calculating the ratio of the light intensity emitted by the acceptor protein CXCR4-GFP 2 (measured at 515±20 nm) over the light intensity emitted by the donor protein CXCR4-Rluc (400±70 nm). The BRET ratio for each experimental condition was expressed over the BRET ratio obtained for mock-treated cells. All the measurements were corrected by subtracting the background BRET signal detected when Rluc-pcDNA vector was expressed alone. Immunogold labelling, replica preparation and electron microscopy analysis Immunogold-labelled cell surface replicas were obtained as described previously [27] , [28] . In brief, Jurkat cells transiently expressing ACP-CXCR4 were stimulated for 30 min at 37 °C with 15 nM CXCL12, 1.5 μM SgG2 or SgG2:CXCL12 at a 100:1 molar ratio, fixed and labelled on ice with an anti-CXCR4 monoclonal antibody (BD Pharmingen) or an isotype control antibody (BD Pharmingen). Afterwards, cells were incubated with protein A conjugated to 10 nm gold particles (Cell Microscopy Center), and attached to mica strips. For the preparation of cell surface replicas by the label-fracture technique, samples were plunge frozen in liquid propane, and then mounted on the sample table of a Balzers400T freeze fracture (FF) unit under liquid nitrogen. The samples were placed in the FF unit, cooled at −150 °C and etched for 12 min to remove excess of ice, and the stage temperature was modified from −150 °C to −90 °C. The samples were shaded with platinum (2 nm at 45 °C angle) and coated with carbon (20 nm at 90 °C angle), removed from the FF unit and floated overnight on a domestic bleach solution to remove the organic material. The replicas were extensively washed in distilled water, mounted on 400 mesh copper grids and examined on a JEM1010 electron microscope (Jeol, Japan) operating at 80 kV. Images were taken at × 10,000 magnification (TemCam-F416 Camera). Overlapping photos of each cell replica were merged with TVIPS software and gold particles were counted using Cell Counter plugin from Image J software. Video microscopy HEK-293T cells were seeded on glass-bottom petri dishes (MatTek cultureware) coated with poly- D -lysine (Sigma). Opti-MEM serum-free medium (Gibco) was used during the assay. HEK-293T cell images shown in Fig. 2 , Fig. 5c and Supplementary Fig. 2 , as well as movies shown in Supplementary Movies 1 and 2 were obtained using a Leica DI6000 microscope stand connected to a SP5 scan head equipped with a temperature-controlled chamber (Cube, LIS, Basel). Images and videos were processed using Image J software. Immunofluorescence For confocal microscopy, the cells were attached to poly- D -lysine-treated coverslips. After stimulation with the chemokine, the vCKBPs or the combination or both at the ratio indicated in each assay, the cells were PFA-fixed and incubated with PBS containing 2% FBS and 2% BSA. The incubation with the primary or secondary Alexa-conjugated antibodies was routinely performed at 37 °C for 1 h or 45 min, respectively. The cells were incubated during 15 min at RT with DAPI reagent (Merck) or FITC-conjugated cholera toxin β (Sigma) when needed. Coverslips were mounted with Prolong Gold antifade mounting medium (Invitrogen). Images were taken by an AxioImager M2 microscopy system coupled to a confocal LSM710 (Zeiss), using × 63 and × 100 PlanApochromat oil immersion objective lens (1.4 numerical aperture) unless indicated. In all the cases, images were obtained at a resolution of 1,024 × 1,024 pixels. The images were subjected to background and mean filter correction using Image J 1.45 software. All co-localization analyses were perfomed using the intensity correlation method (ICA) detailed below. Quantification of co-localization Pearson’s coefficient (PC) is a standard statistical analysis designed to measure the strength of a linear relationship between two variables; in this case, fluorescent intensities from two images. PC generates a range of values from 1, a perfect positive correlation, to −1, a perfect but inverse correlation, with 0 representing a random distribution. To perform a more detailed analysis, we took advantage of a recently developed correlation method termed ICA [57] . The ICA method is based on the principle that if two proteins are part of the same complex then their staining intensities should vary in synchrony, whereas if they form a part of different complexes or structures they will exhibit asynchronous staining. ICA analysis involves generating scatter-plots of stain A or stain B against the product of the difference of each pixel A and B intensities from their respective means. The resulting plots emphasize the high-intensity stained pixels and allow us to identify protein pairs that vary in synchrony, randomly or independently within the cell. The intensity correlation quotient was used to provide an overall index of whether the staining intensities are associated in a random, a dependent or a segregated manner. The outlining of regions in which two probes may distribute is essential to obtain accurate measurements of co-localization [58] . Therefore regions of interest were drawn when necessary. A minimum of three different sections were quantified in the assays shown. Statistical analysis The significant value ( P value) was calculated using GraphPad Prism. How to cite this article: Martinez-Martin, N. et al . Herpes simplex virus enhances chemokine function through modulation of receptor trafficking and oligomerization. Nat. Commun. 6:6163 doi: 10.1038/ncomms7163 (2015).